A selenium-catalysedpara-amination of phenols Antioxidant enzyme glutathione peroxidase (GPx) decomposes hydroperoxides by utilizing the different redox chemistry of the selenium and sulfur. Here, we report a Se-catalysed para -amination of phenols while, in contrast, the reactions with sulfur donors are stoichiometric. A catalytic amount of phenylselenyl bromide smoothly converts N -aryloxyacetamides to N -acetyl p -aminophenols. When the para position was substituted (for example, with tyrosine), the dearomatization 4,4-disubstituted cyclodienone products were obtained. A combination of experimental and computational studies was conducted and suggested the weaker Se−N bond plays a key role in the completion of the catalytic cycle. Our method extends the selenium-catalysed processes to the functionalisation of aromatic compounds. Finally, we demonstrated the mild nature of the para -amination reaction by generating an AIEgen 2-(2′-hydroxyphenyl)benzothiazole (HBT) product in a fluorogenic fashion in a PBS buffer. Selenium is an essential biological trace element discovered by Jöns Jacob Berzelius in 1818 [1] . The selenium analogue of cysteine, known as selenocysteine [2] , [3] , [4] (Sec), is the main biological form of selenium. The most studied selenoenzyme glutathione peroxidase (GPx) has an Sec residue in its active site that is responsible for decomposing hydroperoxides (Fig. 1 a) [5] , [6] . Besides, the flavin-containing redox enzyme thioredoxin reductase (TrxR) [7] , [8] , [9] and the deiodinating enzyme iodothyronine deiodinase (ID) [10] , [11] represent other key selenium-containing enzymes in biocatalysis. Fig. 1 Selected biological reaction and organic reactions catalysed by selenium. a Proposed catalytic cycle of glutathione peroxidase (GPx) for the reduction of hydroperoxides in biology. b Previous reports on organoselenium-catalysed amination of alkenes. GS − glutathione. c Our double [2,3]-sigmatropic rearrangement to achieve para -amination of phenols Full size image Selenium-containing small molecules, such as ebselen and its analogues, have also exhibited important antioxidant activity as GPx mimics [12] , [13] , [14] , [15] . Organoselenium-catalysed reactions have been widely employed in a number of different reactions [16] , [17] , [18] , and substantial progress has been made by Breder [19] , [20] , [21] , Wirth [22] , [23] , [24] , Denmark [25] , [26] , Yeung [27] and Zhao [28] , [29] , [30] , [31] in recent years. Notably, selenium has emerged as appropriate alternatives to precious metals as catalysts for the construction of C–N bonds [32] , [33] , [34] . Breder et al. discovered an elegant selenium-catalysed amination of allyl and vinyl using N -fluorobenzenesulfonimide as oxidant and nitrogen source [35] . Furthermore, Zhao et al. accomplished a powerful pyridination of 1,3-dienes using (BnSe) 2 as a catalyst [36] (Fig. 1b ). However, no selenium-catalysed processes for the functionalisation of aromatic compounds have been developed. One challenge might be the electrophilic selenium catalysts react with the aryl rings directly, leading to the deactivation of catalyst [37] , [38] . We thought that a more nucleophilic site, to accommodate with selenium catalyst temporarily, might be helpful for competing with the deactivation. We herein report a strategy to first form an intermediate with an adjacent, redox versatile Se–N bond which undergoes two successive sigmatropic rearrangements to generate the para -amination product and regenerate the selenium catalyst (Fig. 1c ). Model reactions and substrate scope We started by treating N -phenoxyacetamide ( 1a ) with 1.0 equiv. of N -phenylselanylphthalimide ( C1 ); we observed the para -aminated phenol ( 2a , acetaminophen) in 47% yield. 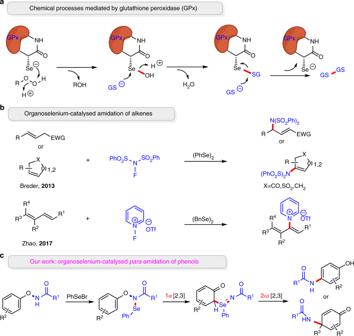Fig. 1 Selected biological reaction and organic reactions catalysed by selenium.aProposed catalytic cycle of glutathione peroxidase (GPx) for the reduction of hydroperoxides in biology.bPrevious reports on organoselenium-catalysed amination of alkenes. GS−glutathione.cOur double [2,3]-sigmatropic rearrangement to achievepara-amination of phenols To our delight, when catalytic amount of C1 (10 mol%) was used, 2a can be obtained in 38% yield (Supplementary Table 1 , entries 1−3). This result compelled us to explore other organoselenium reagents that might catalyse this reaction. No product was detected when diphenyl diselenide ( C2 ) and diphenylselane ( C3 ) were used (Supplementary Table 1 , entries 4 and 5). Both PhSeCl ( C4 ) and PhSeBr ( C5 ) proved to be efficient catalysts in 2,2,2-trifluoroethanol (TFE) with 60 and 79% yields, respectively (Supplementary Table 1 , entries 6 and 7). Screening of a variety of solvents (including MeOH, DMSO, THF, MeCN, EA) indicated that 1,4-dioxane was the best solvent (93% NMR yield and 90% isolated yield of the desired product, Supplementary Table 1 , entries 8−13). Ultimately, the optimal reaction conditions employed 10 mol% PhSeBr ( C5 ) in 1,4-dioxane at room temperature in air. The optimized reaction conditions proved to be effective with a number of other substituents on N -phenoxyacetamides (Table 1 ). N -phenoxyacetamides with electron-rich or electron-deficient substituents reacted smoothly to give the desired para -C–H amination products ( 2a−k ) in moderate to excellent yields (62−92%). Electronic effects did not significantly influence the outcomes of the reactions. N -phenoxyacetamides bearing fluoro-, bromo-, and chloro-substituents ( 2d−e, 2g−h, 2j ) were successfully subjected to this simple protocol with yields from 62 to 83%. The reaction condition was applicable to yield aminated naphthol ( 2l ) in 54% yield. Table 1 Substrate scope of Se-catalysed para -amination of phenols a Full size table To further expand the scope of this highly para -selective amination process, we investigated different N -phenoxyamides. N -phenoxyamide with the Boc-substituent on nitrogen afforded the corresponding product 2m in 76% yield. When the acetyl group was replaced by other aliphatic groups such as cyclopropanecarbonyl and hexanoyl groups, the reactions proceeded smoothly to afford the desired products 2n and 2o in 85 and 53% yield, respectively. Replacing the acetyl group with aromatic amides or sulfonamide also furnished the desired phenols ( 2p − t ) in good yields (64−87%). When we applied the method to the late-stage modification of an antifungal drug Triclosan, the desired para -aminated product ( 2u ) was isolated successfully in 83% yield. 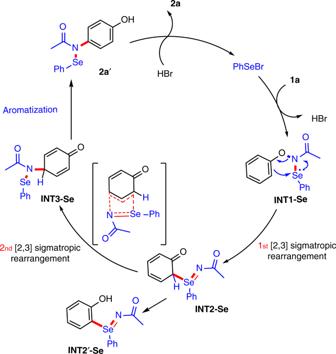Fig. 2 Proposed catalytic cycle of the organoselenium-catalysedpara-amination of phenols. A plausible mechanism illustrating how2ais formed via two consecutive [2,3]-sigmatropic rearrangements The oxidative amination/dearomatization reaction When the para -methyl-substituted substrate was employed, we obtained the dearomatization product 3a in 78% yield (Table 2 ). Efficient oxidative amination of phenols was also obtained when ethyl, propyl was present at the para site under standard reaction condition. However, we did not detect any of the dienones when methyl was replaced with bulkier substituents, such as isopropyl and tert- butyl groups. In those cases, only the corresponding phenols were isolated. Replacing the acetyl group with the propionyl or isobutyryl group on nitrogen gave 3f and 3g in 80 and 61% yield, respectively. Finally, protected tyrosine underwent oxidative amination to give 3h in 56% yield under standard conditions. Table 2 Substrate scope of Se-catalysed dearomatization reaction a Full size table The stoichiometric sulfur-mediated reaction The success in the Se-catalysed synthesis of p -aminophenols or dienones prompted us to attempt to develop a similar sulfur-catalysed version which could display good catalytic activity as organochalcogen catalysis [39] , [40] , [41] , [42] , [43] . However, when a solution of 1a was treated with 10 mol% 2-( p -tolylthio)isoindoline-1,3-dione ( 4a ) at ambient temperature over a period of 5 h, we detected a trace amount of para -aminated product ( 5a ) with a preserved N − S bond. When the amount of 4a was increased to 1.2 equiv., para -aminated product ( 5a ) was obtained in 38% yield. An extensive screening of bases (e.g. pyridine, CsOAc, 2,6-lutidine, DMAP, Na 2 CO 3 , DBU, DIPEA) was conducted and revealed that 2,6-lutidine gave the desired para -aminated product 5a in 53% yield. Further optimization established TFE as the best solvent for this transformation, providing the para -aminated phenol in 84% isolated yield (Supplementary Table 2 ). 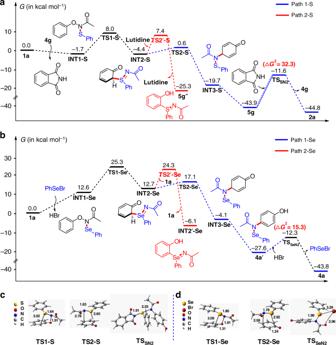Fig. 3 Computational studies on S (and Se)-mediatedpara-selective nitrogen migration ofN-phenoxyacetamide (1a).aComputed Gibbs energy profile for S-mediated reaction (in TFE).bComputed Gibbs energy profile for Se-catalysed reaction (in 1,4-dioxane).cTransition states involved in S-mediated reaction.dTransition states involved in Se-catalysed condition 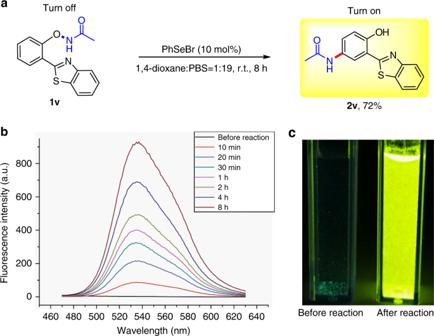Fig. 4 Application of the Se-catalysed reaction in aqueous conditions.aConditions:1v(0.1 mmol), PhSeBr (10 mol%), DMSO/PBS buffer = 1:19 (4.0 mL); at ambient temperature for 8 h; the yield was isolated yield.bFluorescence spectra of reaction in aqueous conditions,λex= 380 nm.cVisual fluorescence of the reaction mixture under a 365 nm ultraviolet lamp With the optimal reaction conditions established, we investigated a series of N -phenoxyacetamide substrates (Table 3 ). Ortho -substituted N- phenoxyacetamides delivered the desired para -aminated phenols in good to excellent yields ( 5a–5c ). When the N -protecting group was replaced by other aliphatic amides such as cyclopropanecarbonyl and propionyl groups, the reactions proceeded smoothly to afford desired products 5e and 5f in 45 and 80% yield, respectively. The reaction proceeded smoothly with both substrates bearing electron-donating group ( 5h ) and halogen-containing N -substituted phthalimides ( 5i–m ). Table 3 Substrate scope of S-mediated reaction a Full size table Mechanistic study A series of experiments were conducted to probe the reaction mechanism. The ortho -sulfiliminyl phenol 5g″ could not transfer to para- aminated product 5g under standard reaction conditions (Supplementary Fig. 1a ). We could not detect any desired product and most of the starting material was recovered when N -methyl-substituted phenoxyacetamide ( 1w ) was used under the S/Se-mediated reaction conditions, indicating the indispensable role of the N–H bond (Supplementary Fig. 1b ). When compounds 1a and d 8 - 1a were used as substrates under S-mediated reaction conditions, the HRMS data showed that the para amide transfer via an intramolecular pathway and the mixed acetamide migration products were not detected. In addition, a crossover experiment was carried out between equimolar amount of 1a and d 8 - 1a under Se-catalysed reaction conditions in one reactor. Only the intramolecular amides transformation of phenols ( 2a , d 7 - 2a ) were obtained (Supplementary Fig. 1c and Supplementary Fig. 13 ). Based on the preliminary studies, the mechanism of this organoselenium-catalysed para -selective C–H bond amination is proposed in Fig. 2 . The electrophilic Se species could react with the mildly basic N -phenoxyacetamide 1a to give the Se–N intermediate ( INT1-Se ) together with the release of one molecule of HBr. Then, the INT1-Se undergoes two successive [2,3]-sigmatropic rearrangements [44] , [45] , [46] , [47] , [48] , [49] to generate the para -amination intermediate ( INT3-Se ), which may readily react with HBr and then rearomatize to the desired product 2a (for details see Supplementary Figs 4 – 11 ). Fig. 2 Proposed catalytic cycle of the organoselenium-catalysed para -amination of phenols. A plausible mechanism illustrating how 2a is formed via two consecutive [2,3]-sigmatropic rearrangements Full size image DFT calculations We performed density functional theory (DFT) calculations to explore the mechanistic details for these S (and Se)-mediated para -selective nitrogen migration of N -aryloxyacetamides (Fig. 3 ). All calculations were carried out with the B3LYP functional [50] , [51] , augmented with Grimmes D3 dispersion correction [52] , [53] , which already proved to be a good choice for chalcogen-containing systems [54] , [55] . For S-mediated reaction, the reaction between N -phenoxyacetamide 1a and N -phenylthiophthalimide 4g was used as model reaction. The Gibbs energy profile is shown in Fig. 3a . First, the reaction of N -phenylthiophthalimide 4g and 1a generates the S–N intermediate INT1-S . Then, the [2,3]-sigmatropic rearrangement of INT1-S via TS1-S forms an ortho -S = N substituted dearomatized species INT2-S , with a barrier of 9.7 kcal mol −1 . Subsequently, the second [2,3]-sigmatropic rearrangement of INT2-S yields the para -amination intermediate INT3-S via TS2-S (with a barrier of 5.0 kcal mol −1 , see path 1-S ). Finally, the aromatization of INT3-S generates the desired product 5g . The whole process is exothermic by 43.9 kcal mol −1 , which indicates that the formation of 5g is reasonable. However, the barrier for the regeneration of N -phenylthiophthalimide 4g (via TS SN2 ) is up to 32.3 kcal mol −1 , suggesting the turnover of 4g is difficult even under basic condition. Therefore, for S-mediated reactions, a stoichiometric amount of N -phenylthiophthalimide is required (see Supplementary Fig. 8 for details). For the Se-catalysed reaction, the Gibbs energy profile of the reaction of 1a and PhSeBr is shown in Fig. 3b . Although the reaction of PhSeBr and 1a generating the Se–N intermediate INT1-Se is endothermic by 12.6 kcal mol −1 , INT1-Se may readily undergo a Se-centred [2,3]-sigmatropic rearrangement to generate an ortho -Se = N substituted dearomatized species ( INT2-Se ) via TS1-Se , with a barrier of 12.7 kcal mol −1 . Then, another N -centred [2,3]-sigmatropic rearrangement of INT2-Se forms para -amination intermediate INT3-Se via TS2-Se (with a barrier of 4.4 kcal mol −1 , see path 1-Se ). Rearomatization of INT3-Se and regeneration of the active catalyst (PhSeBr) from 2a′ affords product 2a readily with large Gibbs energy-driven forces (23.5 and 16.2 kcal mol −1 , respectively). In contrast to N -phenylthiophthalimide, the regeneration of PhSeBr is strongly exothermic by 14.7 kcal mol −1 with a barrier of only 15.3 kcal mol −1 (for details see Supplementary Fig. 11 ). Therefore, PhSeBr could be used as a catalyst. In addition to path 1 , the direct rearomatization of INT2 via TS2′ to generate the ortho -S/Se = N substituted phenol ( INT2′ ) is also possible (see path 2-S in Fig. 3a and path 2-Se in Fig. 3b ). However, the activation barriers of path 2 in these two systems are much higher than that of path 1 . The calculated trends for the two reactions are consistent with the fact that no ortho -Se = N substituted phenol (or only small amount of ortho -S = N substituted phenol) was obtained for these two types of reactions. Therefore, path 1 involving two successive [2,3]-sigmatropic rearrangements is mainly responsible for the two para -selective amination reactions (for details see Supplementary Figs 2 – 11 and Supplementary Data 1 ). Fig. 3 Computational studies on S (and Se)-mediated para -selective nitrogen migration of N- phenoxyacetamide ( 1a ). a Computed Gibbs energy profile for S-mediated reaction (in TFE). b Computed Gibbs energy profile for Se-catalysed reaction (in 1,4-dioxane). c Transition states involved in S-mediated reaction. d Transition states involved in Se-catalysed condition Full size image Synthetic application To further explore the mild nature of our method, an HBT-substrate 1v was subjected to the reaction condition in a mixed solvent of 95% PBS buffer and 5% 1,4-dioxane (Fig. 4a ). The obtained product 2v exhibits significant aggregation-induced emission behaviours [56] , [57] , [58] , [59] , [60] . The fluorescence intensity of the product increased gradually at 538 nm (Fig. 4b ) in the reaction solution, accompanied by a dramatic change in emission colour from pale blue to bright yellow (Fig. 4c ). Fig. 4 Application of the Se-catalysed reaction in aqueous conditions. a Conditions: 1v (0.1 mmol), PhSeBr (10 mol%), DMSO/PBS buffer = 1:19 (4.0 mL); at ambient temperature for 8 h; the yield was isolated yield. b Fluorescence spectra of reaction in aqueous conditions, λ ex = 380 nm. c Visual fluorescence of the reaction mixture under a 365 nm ultraviolet lamp Full size image In summary, we discovered an organoselenium-catalysed para -amination of phenols or dienones under mild conditions. The methodology features a broad substrate scope and a high para -selectivity. More importantly, this work reveals a significant difference between the sulfenylation reagents and organoselenium reagents. While experimental and computational studies suggest that both the sulfur and selenium variants proceed through a double [2,3]-sigmatropic rearrangement, the sulfenylation reagents behave as coupling partners while organoselenium reagents can be employed catalytically. Because of the larger atomic radius of selenium compared to sulfur, selenium is more polarizable (“softer”) than sulfur, allowing intrinsic selenium to be more nucleophilic and electrophilic [61] , [62] . Compared to sulfur, the larger hybridized orbitals of selenium results in weaker σ overlap [63] . So most bond strength of Se−X is weaker. The differences between sulfur and selenium developed here are reminiscent of their behaviours in biology. For example, the catalytic activity of the native enzyme dramatically reduces when the Sec residue in the type I ID enzyme was replaced by a cysteine (Cys) moiety [64] , [65] . We expect our present work to stimulate future studies of selenium as an alternative catalytic platform to transition metal-catalysed C–H amination reactions. Materials For NMR spectra of compounds in this manuscript, see Supplementary Figs 14 – 73 . For the crystallographic data of compound 2n and 5a , see Supplementary Fig. 12 and Supplementary Tables 3 – 15 . For the representative experimental procedures and analytic data of compounds synthesized, see Supplementary Methods. Se-catalysed standard reaction conditions N -phenoxyamides ( 1 ) (0.20 mmol), PhSeBr (10 mol%), were weighed into a 10 mL tube, to which was added 1,4-dioxane (2.0 mL). The reaction vessel was stirred at room temperature for 8 h. Then the mixture was concentrated under vacuum and the residue was purified by column chromatography on silica gel with a gradient eluent of petroleum ether and ethyl acetate to afford the corresponding product 2 or 3 . S-mediated standard reaction conditions N -phenoxyacetamides ( 1 ) (0.20 mmol), N -substituted thiophthalimides ( 4 ) (0.24 mmol) and 2,6-lutidine (1.0 eq.) were weighed into a 10 mL tube, to which was added TFE (2.0 mL). The reaction vessel was stirred at room temperature for 5 h in air. The mixture was then concentrated under vacuum and the residue was purified by column chromatography on silica gel with a gradient eluent of petroleum ether and ethyl acetate to afford the corresponding product ( 5 ).